SUMO modification of the neuroprotective protein TDP1 facilitates chromosomal single-strand break repair Breaking and sealing one strand of DNA is an inherent feature of chromosome metabolism to overcome torsional barriers. Failure to reseal broken DNA strands results in protein-linked DNA breaks, causing neurodegeneration in humans. This is typified by defects in tyrosyl DNA phosphodiesterase 1 (TDP1), which removes stalled topoisomerase 1 peptides from DNA termini. Here we show that TDP1 is a substrate for modification by the small ubiquitin-like modifier SUMO. We purify SUMOylated TDP1 from mammalian cells and identify the SUMOylation site as lysine 111. While SUMOylation exhibits no impact on TDP1 catalytic activity, it promotes its accumulation at sites of DNA damage. A TDP1 SUMOylation-deficient mutant displays a reduced rate of repair of chromosomal single-strand breaks arising from transcription-associated topoisomerase 1 activity or oxidative stress. These data identify a role for SUMO during single-strand break repair, and suggest a mechanism for protecting the nervous system from genotoxic stress. Mutation of tyrosyl DNA phosphodiesterase 1 (TDP1) underlies the demise of postmitotic neurons observed in the human genetic neurological disease Spinocerebellar Ataxia with Axonal Neuropathy [1] . In budding yeast, TDP1 operates at DNA double-strand breaks (DSBs) primarily created by collision of replication forks with topoisomerase 1 (Top1) intermediates in proliferating cells [2] , [3] . In higher organisms, TDP1 additionally operates at single-strand breaks (SSBs), independently of DNA replication [4] , [5] , [6] . TDP1-deficient mammalian cells and postmitotic neurons display reduced rates of repairing SSBs arising from Top1 activity, hydrogen peroxide or ionizing radiation (IR) [1] , [4] , [5] , [7] , [8] . TDP1 also processes a variety of damaged 3′-termini such as 3′-phosphoglycolate and 3′-abasic sites [7] , [9] , [10] , [11] , [12] , [13] , [14] , [15] . Although defects in TDP1 lead to accumulation of SSBs, cell-free studies suggest a requirement of high local concentrations of TDP1 to repair these structures [16] . However, it is not clear how this regulation is achieved in cells. Post-translational modifications have been implicated in modulating the function of several DNA repair factors and channel repair to specific pathways. For example, phosphorylation of TDP1 by ATM or DNA-PK has been shown to promote its function at DSBs [17] , [18] . Phosphorylation by ATM during DSB repair has also been shown to promote the activity of polynucleotide kinase phosphatase [19] . Here we identify TDP1 as a target for modification by the small ubiquitin-like modifier SUMO and provide evidence implicating SUMOylation in facilitating TDP1 cellular function during SSB repair. TDP1 is a substrate for modification by SUMO Yeast two-hybrid analyses conducted to identify novel TDP1 binding partners uncovered 14 independent clones encoding full-length UBE2I, the human homologue of the yeast SUMO-conjugating enzyme UBC9 ( Fig. 1a ). These observations suggested a previously unanticipated role for the SUMO modification pathway during TDP1-mediated repair. To test whether TDP1 is a substrate for covalent SUMO conjugation, we first reconstituted SUMOylation reactions in vitro using recombinant human p53, a known SUMO target [20] ( Fig. 1b ). Parallel reactions conducted with human recombinant TDP1 revealed a slower migrating band, as detected by anti-TDP1 or anti-SUMO1 antibodies ( Fig. 1c ). These products were absent from control reactions conducted in the presence of a SUMO1 mutant that is incapable of forming the covalent conjugation reaction. Furthermore, their appearance was dependent on ATP ( Fig. 1d ), confirming that they are covalent TDP1–SUMO1 conjugates. Subsequent comparison of the different SUMO isoforms suggested that TDP1 is preferentially modified by SUMO1 ( Fig. 1e ). As most SUMO target proteins are modified at very low steady-state levels in vivo , we ectopically expressed TDP1 and SUMO1 in mammalian cells and examined the possibility of covalent TDP1–SUMO1 conjugations. For these experiments, we transfected HEK293 cells with Myc–TDP1 and/or green fluorescent protein (GFP)–SUMO1, followed by immunoprecipitation using anti-Myc antibodies. Probing the immunoprecipitate (IP) with anti-Myc antibodies revealed a discrete slower migrating band in Myc–IPs from extracts coexpressing Myc–TDP1 and GFP–SUMO1 ( Fig. 1f ). Importantly, this band was absent in Myc–IPs conducted on extracts expressing either Myc–TDP1 or GFP–SUMO1 alone. Furthermore, probing with anti-SUMO1 antibodies revealed a faint band in the input of extracts coexpressing Myc–TDP1 and GFP–SUMO1, but not in extracts expressing either Myc–TDP1 or GFP–SUMO1 alone. Enrichment of this band was observed following Myc–IPs, confirming that it is a TDP1–SUMO1 modification. Parallel experiments conducted using SUMO1, SUMO2 or SUMO3 isoforms were in agreement with the in vitro observations, suggesting that while TDP1 can be modified by all three SUMO isoforms its primary substrate appears to be SUMO1 ( Fig. 1g ). 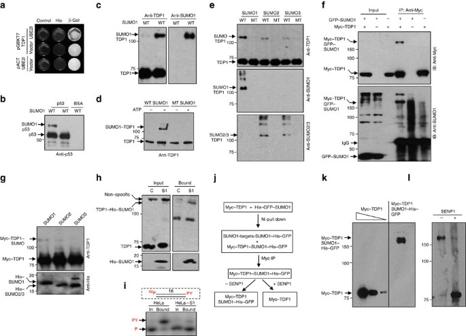Figure 1: Human TDP1 is SUMOylatedin vitroand in mammalian cells. (a) Yeast Y190 cells containing the indicated constructs were examined for the activation ofHis3andβ-Galreporter genes. (b) Recombinant p53 (430 nM) was incubated with 50 nM SAE1/SAE2, 500 nM UBC9, 5 mM ATP and 30 μM SUMO1 'WT' or mutant SUMO1 that cannot be covalently conjugated 'MT'. Reactions were fractionated by SDS–PAGE and analysed by anti-p53 immunoblotting (Activemotif). (c) Human full-length TDP1 (500 nM) was subjected toin vitroSUMOylation reactions and analysed by anti-TDP1 (ab4166; Abcam) or anti-SUMO1 (Santa Cruz, SC-5308) immunoblotting. (d) SUMOylation reactions were conducted in the presence or absence of 5 mM ATP. (e) SUMOylation reactions conducted in the presence of SUMO1, SUMO2 or SUMO3 were divided into three fractions and analysed by immunoblotting. (f) Total cell extract from HEK293 (∼4×106cells) transfected with Myc–TDP1 and/or GFP–SUMO1 was subjected to immunoprecipitation using anti-Myc monoclonal antibodies (9B11; Cell Signaling). Immunoprecipitates were analysed by immunoblotting using anti-Myc (9B11) or anti-SUMO1 (SC-5308) antibodies. Input is∼5% of total cell extract. (g) HEK293 cells transfected with Myc–TDP1, HA-tagged His–SUMO1, His–SUMO2 or His–SUMO3 were analysed by anti-TDP1 (ab4166) or anti-His (H1029) immunoblotting. (h) Lysates from control HeLa cells 'C' or cells stably expressing His–SUMO1 'S1' were mixed with Ni2+charged agarose beads and histidine-tagged SUMO conjugates 'bound' were analysed by anti-TDP1 immunoblotting. Input is∼3% of total cell extract. (i) Total cell extract 'In' (∼20 μg) or Ni2+beads enriched with histidine-tagged SUMO conjugates 'bound' were mixed with32P-radiolabelled 18-mer duplex (50 nM) harbouring a 3′-phosphotyrosine terminus 'PY', inset. Repair products were analysed by denaturing PAGE and phosphorimaging. Positions of the32P-radiolabelled substrate 'PY' and product 'P' are indicated. (j) Diagram depicting purification of SUMOylated TDP1 from mammalian cells. (k) Serial dilutions of purified Myc–TDP1 or Myc–TDP1–SUMO1–His–GFP were analysed by SDS–PAGE and anti-Myc immunoblotting. (l) Purified Myc-TDP1–SUMO1–His–GFP was mock-treated '−' or incubated with 250 ng of human sentrin/SUMO-specific protease-1 (SENP1) '+' and reaction products analysed by anti-Myc immunoblotting. Molecular weight size markers (kDa) are depicted. IB, immunoblot; IgG, immunoglobulin G; MT, mutant; WT, wild type. Figure 1: Human TDP1 is SUMOylated in vitro and in mammalian cells. ( a ) Yeast Y190 cells containing the indicated constructs were examined for the activation of His3 and β-Gal reporter genes. ( b ) Recombinant p53 (430 nM) was incubated with 50 nM SAE1/SAE2, 500 nM UBC9, 5 mM ATP and 30 μM SUMO1 'WT' or mutant SUMO1 that cannot be covalently conjugated 'MT'. Reactions were fractionated by SDS–PAGE and analysed by anti-p53 immunoblotting (Activemotif). ( c ) Human full-length TDP1 (500 nM) was subjected to in vitro SUMOylation reactions and analysed by anti-TDP1 (ab4166; Abcam) or anti-SUMO1 (Santa Cruz, SC-5308) immunoblotting. ( d ) SUMOylation reactions were conducted in the presence or absence of 5 mM ATP. ( e ) SUMOylation reactions conducted in the presence of SUMO1, SUMO2 or SUMO3 were divided into three fractions and analysed by immunoblotting. ( f ) Total cell extract from HEK293 ( ∼ 4×10 6 cells) transfected with Myc–TDP1 and/or GFP–SUMO1 was subjected to immunoprecipitation using anti-Myc monoclonal antibodies (9B11; Cell Signaling). Immunoprecipitates were analysed by immunoblotting using anti-Myc (9B11) or anti-SUMO1 (SC-5308) antibodies. Input is ∼ 5% of total cell extract. ( g ) HEK293 cells transfected with Myc–TDP1, HA-tagged His–SUMO1, His–SUMO2 or His–SUMO3 were analysed by anti-TDP1 (ab4166) or anti-His (H1029) immunoblotting. ( h ) Lysates from control HeLa cells 'C' or cells stably expressing His–SUMO1 'S1' were mixed with Ni 2+ charged agarose beads and histidine-tagged SUMO conjugates 'bound' were analysed by anti-TDP1 immunoblotting. Input is ∼ 3% of total cell extract. ( i ) Total cell extract 'In' ( ∼ 20 μg) or Ni 2+ beads enriched with histidine-tagged SUMO conjugates 'bound' were mixed with 32 P-radiolabelled 18-mer duplex (50 nM) harbouring a 3′-phosphotyrosine terminus 'PY', inset. Repair products were analysed by denaturing PAGE and phosphorimaging. Positions of the 32 P-radiolabelled substrate 'PY' and product 'P' are indicated. ( j ) Diagram depicting purification of SUMOylated TDP1 from mammalian cells. ( k ) Serial dilutions of purified Myc–TDP1 or Myc–TDP1–SUMO1–His–GFP were analysed by SDS–PAGE and anti-Myc immunoblotting. ( l ) Purified Myc-TDP1–SUMO1–His–GFP was mock-treated '−' or incubated with 250 ng of human sentrin/SUMO-specific protease-1 (SENP1) '+' and reaction products analysed by anti-Myc immunoblotting. Molecular weight size markers (kDa) are depicted. IB, immunoblot; IgG, immunoglobulin G; MT, mutant; WT, wild type. Full size image Next, we tested whether endogenous TDP1 is covalently conjugated by SUMO1. For these experiments, we used HeLa cells stably expressing hexahistidine (6×His)-tagged SUMO1. We purified histidine-tagged SUMO conjugates using nickel-charged beads and subjected the conjugation products to immunoblotting using anti-TDP1 antibodies. Endogenous TDP1–SUMO1 was enriched on nickel beads incubated with extracts expressing histidine-tagged SUMO1, but not with control HeLa cell extracts ( Fig. 1h ). That the enriched products correspond to TDP1–SUMO1 conjugates was confirmed by demonstrating TDP1 activity that releases tyrosine from a 3′-phosphotyrosine synthetic Top1 substrate, which mimics Top1-linked DNA breaks ( Fig. 1i ). To further confirm that TDP1 is covalently SUMOylated in mammalian cells, we examined the effect of sentrin/SUMO-specific protease-1 (SENP1) on human purified SUMO1–TDP1 conjugates. SUMOylation is a dynamic process and once attached the SUMO peptide can be removed from target proteins by SENPs. For these experiments, we transfected HEK293 cells with His–GFP–SUMO1 and/or Myc–TDP1 and purified histidine-tagged GFP–SUMO1 conjugate using nickel-charged beads. Conjugation products were then subjected to Myc–IPs to purify Myc–TDP1–SUMO1–His–GFP products ( Fig. 1j ). Anti-Myc immunoblotting revealed a discrete band in Myc–IPs from extracts coexpressing Myc–TDP1 and His–GFP–SUMO1 ( Fig. 1k ). Subsequent treatment of the Myc–IP with SENP1 resulted in a band corresponding in size to Myc–TDP1 ( Fig. 1l ). Taken together, we conclude that TDP1 is covalently modified by SUMO1 in mammalian cells. TDP1 is SUMOylated at lysine 111 To study the consequences of TDP1 SUMOylation, we aimed at identifying SUMOylation site(s). Most SUMO target proteins contain a specific stretch of ψKxE, where ψ is a large hydrophobic residue and K is the target lysine. In silico analyses revealed two potential SUMOylation sites in the N-terminal domain and three sites in the C-terminal domain ( Fig. 2a ). We mutated the predicted acceptor lysines to arginine and subjected the purified proteins to in vitro SUMOylation reactions. Notably, the N-terminal domain is only conserved in higher eukaryotes ( Fig. 2b , dotted boxes) and database analyses revealed K111 to be conserved across vertebrates. Consistent with SUMOylation occurring in this domain, reactions conducted in the presence of TDP1 1−150 revealed a prominent slower migrating band ( Fig. 2c , lane 1). This band was absent from reactions containing TDP1 1−150; K111R and instead a faster migrating band appeared with lower intensity, suggesting a secondary SUMOylation site that was picked up in the absence of K111 in vitro ( Fig. 2c , lane 2). Mutation of K139 to arginine resulted in SUMOylated species with identical size to SUMOylated TDP1 1−150 , albeit with higher intensity, suggesting that K111 is the main SUMOylation site and that K139 may contribute to SUMOylation of the truncated TDP1 1−150 in vitro ( Fig. 2c , lane 3). Indeed, mutation of both K111 and K139 to arginine completely abrogated SUMOylation of TDP1 1−150 ( Fig. 2c , lane 4). The slower migrating band was SUMOylated TDP1, as it was absent in reactions containing a mutant form of SUMO that cannot be covalently conjugated ( Fig. 2c , lanes 5 and 6). We next compared full-length recombinant TDP1 and TDP1 K111R for their ability to covalently conjugate SUMO1 in vitro . Mutation of lysine 111 to arginine was sufficient to abolish SUMO1 covalent attachment to full-length TDP1 ( Fig. 2d ). We next examined whether lysine 111 is the main SUMOylation site in vivo . For these experiments, we generated Myc–TDP1 and mutants in which the N-terminal, C-terminal or all predicted SUMO sites were mutated to arginine ( Fig. 2e ). We co-transfected HEK293 cells with the different forms of Myc–TDP1 and/or GFP–SUMO1, followed by immunoprecipitation using anti-Myc antibodies. A single amino-acid substitution of K111 to arginine was sufficient to abrogate the formation of TDP1–SUMO1 conjugates ( Fig. 2e ). Taken together, we conclude that K111 is the main SUMOylation site in TDP1. 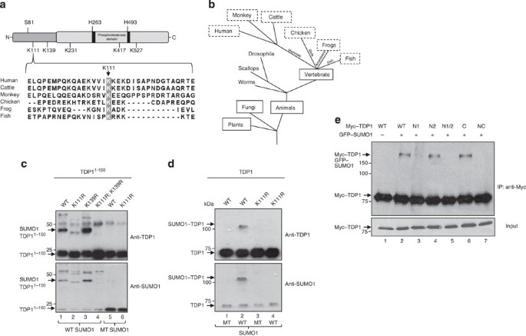Figure 2: TDP1 is SUMOylated at Lysine 111. (a,b) BLAST analysis identifies TDP1 orthologues in plants, fungi and animals with an extended amino terminus in vertebrates 'dotted boxes'. Sequence analysis of this domain identifies two putative SUMOylation sites. Alignment of sequences from human (Homo sapiens; NP_001008744), cattle (Bos taurus; NP_001180084; XP_874680), monkey (Pongo abelii; XP_002825063), chicken (Gallus gallus; XP_421313), frog (Xenopus tropicalis;NP_001039242), fish (Danio rerio; XP_700174) using UniProt software identifies K111 (highlighted in grey) as a conserved residue. (c) Purified human TDP1 encompassing the first 150 amino acids TDP11−150'WT' and equivalent versions, in which lysine 111, 139 or both were mutated to arginine 'K111R, K139R and K111R; K139R, respectively' were subjected to SUMOylation reactions containing 50 nM SAE1/SAE2, 500 nM UBC9 and 5 mM ATP in the presence of 30 μM WT SUMO1 (lanes 1–4) or mutant SUMO1 (lanes 5 and 6). Reaction products were fractionated by SDS–PAGE and analysed by immunoblotting with anti-TDP1 (ab4166; Abcam) or anti-SUMO1 (Activemotif) antibodies. (d) Purified full-length human TDP1 'WT' or TDP1K111R'K111R' was subjected to SUMOylation reactions and analysed by immunoblotting. (e) HEK293 cells were transfected with '+' or without '−' GFP–SUMO1 and with wild-type Myc–TDP1 or a version harbouring substitution of K111 'N1', K139 'N2', K111 and K139 'N1/2', K231, K417 and K527 'C' or K111, K139, K231, K417 and K527 'NC' to arginine. Total cell extract (∼4×106cells) was subjected to immunoprecipitation using anti-Myc monoclonal antibodies (9B11; Cell Signaling) and immunoprecipitates were fractionated by SDS–PAGE and analysed by immunoblotting. Molecular weight size markers (kDa) are depicted. MT, mutant; WT, wild type. Figure 2: TDP1 is SUMOylated at Lysine 111. ( a , b ) BLAST analysis identifies TDP1 orthologues in plants, fungi and animals with an extended amino terminus in vertebrates 'dotted boxes'. Sequence analysis of this domain identifies two putative SUMOylation sites. Alignment of sequences from human ( Homo sapiens; NP_001008744 ), cattle ( Bos taurus; NP_001180084; XP_874680 ), monkey ( Pongo abelii; XP_002825063 ), chicken ( Gallus gallus; XP_421313 ), frog ( Xenopus tropicalis ; NP_001039242 ), fish ( Danio rerio; XP_700174 ) using UniProt software identifies K111 (highlighted in grey) as a conserved residue. ( c ) Purified human TDP1 encompassing the first 150 amino acids TDP1 1−150 'WT' and equivalent versions, in which lysine 111, 139 or both were mutated to arginine 'K111R, K139R and K111R; K139R, respectively' were subjected to SUMOylation reactions containing 50 nM SAE1/SAE2, 500 nM UBC9 and 5 mM ATP in the presence of 30 μM WT SUMO1 (lanes 1–4) or mutant SUMO1 (lanes 5 and 6). Reaction products were fractionated by SDS–PAGE and analysed by immunoblotting with anti-TDP1 (ab4166; Abcam) or anti-SUMO1 (Activemotif) antibodies. ( d ) Purified full-length human TDP1 'WT' or TDP1 K111R 'K111R' was subjected to SUMOylation reactions and analysed by immunoblotting. ( e ) HEK293 cells were transfected with '+' or without '−' GFP–SUMO1 and with wild-type Myc–TDP1 or a version harbouring substitution of K111 'N1', K139 'N2', K111 and K139 'N1/2', K231, K417 and K527 'C' or K111, K139, K231, K417 and K527 'NC' to arginine. Total cell extract ( ∼ 4×10 6 cells) was subjected to immunoprecipitation using anti-Myc monoclonal antibodies (9B11; Cell Signaling) and immunoprecipitates were fractionated by SDS–PAGE and analysed by immunoblotting. Molecular weight size markers (kDa) are depicted. MT, mutant; WT, wild type. Full size image SUMOylation-deficient mutant shows reduced rate of SSB repair To examine the consequences of TDP1 SUMOylation in vivo , we compared the ability of HEK293 cells ectopically expressing SUMO1 and TDP1 or TDP1 K111R for their ability to repair camptothecin (CPT)-induced DNA damage using alkaline comet assays. These assays primarily measure repair of DNA SSBs, where they form and disappear with kinetics established for this repair process [4] , [5] , [21] . As expected, HEK293 cells expressing TDP1 accumulated four- to fivefold fewer SSBs compared with control cells ( Fig. 3a ). Notably, cells expressing TDP1 K111R accumulated two- to threefold more SSBs compared with TDP1-expressing cells ( P =0.0169; t -test). This defect was not due to differences in expression levels as confirmed by immunoblotting ( Fig. 3b ) and was evident from scatter plots of the raw data from individual experiments ( Fig. 3c ). The difference in breaks is notable in terms of SSB repair, as ∼ 4-fold difference underlies the severe neurological demise observed in neural tissues lacking XRCC1, the core SSB repair protein [22] . To examine whether the difference in repair was due to SUMOylation, we compared CPT-induced SSBs in the presence and absence of ectopically expressed SUMO1. While overexpression of SUMO1 had no impact on CPT-induced SSBs in control cells and in TDP1 K111R -expressing cells ( Fig. 3d,e ; P =0.65; t -test), it reduced the extent of SSBs in TDP1-expressing cells ( P =0.007; t -test). These observations suggest that the difference in repair observed between TDP1 K111R and TDP1 was due to SUMOylation of the latter. As TDP1 also repairs oxidative SSBs resulting from IR [23] , we compared TDP1- and TDP1 K111R -expressing cells for their ability to repair IR-induced SSBs. While IR induced similar levels of SSBs in all three cell lines ( Fig. 3f ), the kinetics of their removal was delayed in cells expressing TDP1 K111R compared with TDP1-expressing cells ( Fig. 3g ), suggesting a role for TDP1 lysine 111 during the repair of IR-induced SSBs. 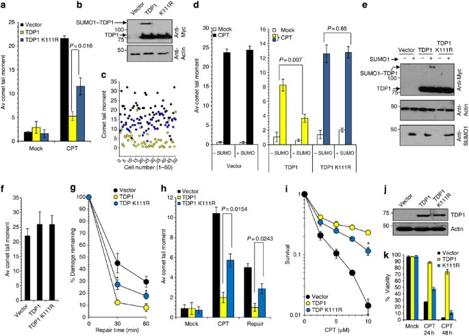Figure 3: The SUMOylation-deficient mutant TDP K111R displays attenuated rate of SSB repair. (a) HEK293 cells were transfected with GFP–SUMO1 and empty vector 'vector', or vectors encoding Myc–TDP1 'TDP1' or Myc–TDP1K111R'TDP1 K111R' using conditions that produce >90% transfection efficiency. Cells were incubated with DMSO 'mock' or 50 μM camptothecin 'CPT' and DNA breaks quantified by alkaline comet assays (ACA). Mean tail moments were quantified for 50 cells per sample per experiment, and data are the average ofn=3 biological replicates±s.e.m. (b) Lysate from cells used inawas analysed by immunoblotting. (c) A representative scatter plot from one experiment showing comet tail moments of 50 individual cells per sample. (d) HEK293 cells transfected with the indicated TDP1 constructs and an empty GFP '−SUMO1' or GFP1–SUMO1 '+SUMO1' vector were analysed by ACA. (e) Lysate from cells used indwere analysed by immunoblotting. (f,g) HEK293 were exposed to ionizing radiation (20 Gy) and DNA breaks quantified immediately following irradiation (f) or after subsequent incubation for the indicated repair periods by ACA (g). The fraction of DNA breaks remaining was calculated fromn=3 biological replicates and depicted as % damage remaining±s.e.m. (h)Tdp1−/−MEFs infected with virus particles encoding vector alone, human TDP1 or human TDP1 K111R were subjected to 20 μM CPT followed by subsequent incubation in CPT-free media for 60 min, and DNA breaks were quantified by ACA. (i)Tdp1−/−MEFs were mock-treated or treated with the indicated doses of CPT, and the number of surviving colonies was calculated fromn=4 biological replicates±s.e.m. (j)Tdp1−/−MEFs lysate from experiments iniwas analysed by immunoblotting. (k)Tdp1−/−primary cortical neural cells electroporated with empty GFP vector or vectors expressing human GFP–TDP1 or GFP–TDP1K111Rwere exposed to 30 μM CPT (4× 30 min pulse every 3 h) and viability of GFP-positive cells quantified using propidium iodide exclusion. Error bars, range of error forn=2 biological replicates. Statistical analyses were conducted using Student'st-test, and asterisks denoteP<0.05 difference between TDP1 (yellow) and TDP1 K111R (blue). Where not visible, error bars are smaller than the symbols. Figure 3: The SUMOylation-deficient mutant TDP K111R displays attenuated rate of SSB repair. ( a ) HEK293 cells were transfected with GFP–SUMO1 and empty vector 'vector', or vectors encoding Myc–TDP1 'TDP1' or Myc–TDP1 K111R 'TDP1 K111R' using conditions that produce >90% transfection efficiency. Cells were incubated with DMSO 'mock' or 50 μM camptothecin 'CPT' and DNA breaks quantified by alkaline comet assays (ACA). Mean tail moments were quantified for 50 cells per sample per experiment, and data are the average of n =3 biological replicates±s.e.m. ( b ) Lysate from cells used in a was analysed by immunoblotting. ( c ) A representative scatter plot from one experiment showing comet tail moments of 50 individual cells per sample. ( d ) HEK293 cells transfected with the indicated TDP1 constructs and an empty GFP '−SUMO1' or GFP1–SUMO1 '+SUMO1' vector were analysed by ACA. ( e ) Lysate from cells used in d were analysed by immunoblotting. ( f , g ) HEK293 were exposed to ionizing radiation (20 Gy) and DNA breaks quantified immediately following irradiation ( f ) or after subsequent incubation for the indicated repair periods by ACA ( g ). The fraction of DNA breaks remaining was calculated from n =3 biological replicates and depicted as % damage remaining±s.e.m. ( h ) Tdp1−/− MEFs infected with virus particles encoding vector alone, human TDP1 or human TDP1 K111R were subjected to 20 μM CPT followed by subsequent incubation in CPT-free media for 60 min, and DNA breaks were quantified by ACA. ( i ) Tdp1 −/− MEFs were mock-treated or treated with the indicated doses of CPT, and the number of surviving colonies was calculated from n= 4 biological replicates±s.e.m. ( j ) Tdp1 −/− MEFs lysate from experiments in i was analysed by immunoblotting. ( k ) Tdp1 −/− primary cortical neural cells electroporated with empty GFP vector or vectors expressing human GFP–TDP1 or GFP–TDP1 K111R were exposed to 30 μM CPT (4× 30 min pulse every 3 h) and viability of GFP-positive cells quantified using propidium iodide exclusion. Error bars, range of error for n =2 biological replicates. Statistical analyses were conducted using Student's t -test, and asterisks denote P <0.05 difference between TDP1 (yellow) and TDP1 K111R (blue). Where not visible, error bars are smaller than the symbols. Full size image To further examine the consequences of TDP1 SUMOylation in cells lacking endogenous TDP1, we infected Tdp1−/− mouse embryonic fibroblasts (MEFs) with retrovirus particles containing vector alone (Tdp1 −/− V ) or encoding human TDP1 (Tdp1 −/− hTDP1 ) or TDP1 K111R (Tdp1 −/− hTDP1−K111R ). During 30-min incubation with CPT, Tdp1 −/− V accumulated approximately fivefold more SSBs compared with cells complemented with wild-type human TDP1, Tdp1 −/− hTDP1 ( Fig. 3h ). Importantly, Tdp1 −/− hTDP1−K111R cells accumulated ∼ 3-fold more breaks compared with Tdp1 −/− hTDP1 cells ( P =0.015; t -test). Consistent with the kinetics of SSB repair, subsequent incubation in CPT-free medium for short periods resulted in a decline in the level of SSBs observed in all three cell lines. Notably, levels of SSBs remained at a higher level in Tdp1 −/− hTDP1−K111R compared with Tdp1 −/− hTDP1 cells. To examine whether unrepaired SSBs in Tdp1 −/− hTDP1−K111R impacted on cellular survival, we compared the three cell types for their ability to form macroscopic colonies following exposure to CPT. Tdp1 −/− V cells were very sensitive to CPT and, as expected, complementation with hTDP1 led to marked protection, whereas complementation with hTDP1 K111R led to partial protection ( Fig. 3i,j ). Furthermore, complementation of Tdp1 −/− quiescent cortical neural cells with human TDP1 or TDP1 K111R revealed a role for K111 to maintain cell viability following CPT ( Fig. 3k ). Taken together, we conclude that mutating the acceptor lysine K111 to a non-SUMOylatable arginine results in defects in repairing SSBs. K111R does not alter TDP1 structure or catalytic activity Why does a TDP1 SUMOylation-defective mutant display attenuated rates of SSB repair? Although unlikely for missense point mutations, we tested the possibility that the K111R mutation might lead to a gross distortion of TDP1 structure. We subjected recombinant TDP1 and TDP1 K111R produced in Escherichia coli to thermal denaturation experiments, a widely used technique to examine structural changes of proteins [24] . The K111R mutation had no detectable impact on the thermal stability or unfolding profile of TDP1, as determined by comparing the denaturation curves and their corresponding melting temperatures ( Fig. 4a ). We also compared the circular dichroism absorption spectrum of TDP1 and TDP1 K111R ( Fig. 4b–d ). The two proteins gave spectral shapes with negative bands at ∼ 210 and 220 nm, and positive bands at ∼ 195 nm. Analyses of secondary structure by the variable selection algorithm (CDSSTR), which provides superior fits for globular proteins [25] , [26] , [27] , [28] , revealed no significant difference in α-helical or β-sheet content ( P >0.5; t -test), suggesting no apparent change in structure ( Supplementary Table S1 ). This was also supported by using the CONTIN and K2D algorithms ( Supplementary Tables S2 and S3 ). To further examine the impact on protein folding and catalytic activity, we incubated purified recombinant TDP1 or TDP1 K111R with oligonucleotide duplexes harbouring 3′-phosphotyrosine that mimic Top1-linked breaks and quantified the 3′-phosphate products. The reactions showed a comparable concentration-dependent conversion of 3′-phosphotyrosine to 3′-phosphate, suggesting no impact of the K111R mutation on catalytic activity ( Fig. 4e,f ). Taken together, we conclude that mutation of the SUMOylation site of TDP1 to a non-SUMOylatable version results in delayed rate of SSB repair without a measurable impact on structure or catalytic activity. 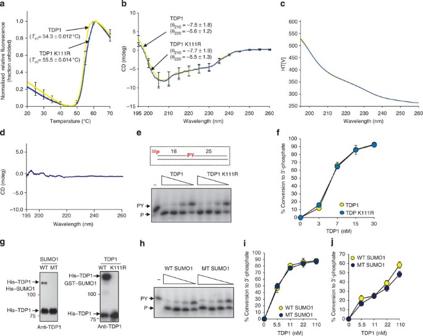Figure 4: The K111R mutation does not result in a measurable change of TDP1 structure or catalytic activity. (a) Recombinant TDP1 or TDP1K111Rwas mixed with SYPRO-Orange, and melting profiles were obtained between 20 and 70 °C using a ramping rate of 0.03 °C s−1. Data were normalized to a fraction of protein in its denatured state and presented as normalized relative fluorescence. Melting temperatures (Tm) were determined according to the Boltzmann model55. Error bars represent s.d. fromn=3 independent replicates. (b,c) Recombinant TDP1 or TDP1K111Rwas placed in a 0.2-mm quartz cuvette and the circular dichroism spectrum determined using a JASCO J-715 spectropolarimeter. Scans were performed from 260 to 195 nm, buffer baselines were subtracted, and data recorded with a high-tension voltage 'HT [V]' <550 V. Data represent the average ofn=4 independent replicates±s.e.m. (d) Subtraction of the TDP1 K111R spectra from that of TDP1 shows no gross structural difference. (e) Decreasing concentrations (30, 15, 7 and 3 nM) of purified recombinant TDP1 or TDP1K111Rwas incubated with a32P-radiolabelled duplex-nicked substrate (50 nM) harbouring a 3′-phosphotyrosine 'PY' at the nick (inset). Repair products were analysed by denaturing PAGE and phosphorimaging. Positions of the32P-radiolabelled substrate 'PY' and product 'P' are indicated by arrows. (f) Reaction products 'P' were quantified relative to total labelled substrate 'P+PY' and percentage conversion to 3′-P from experiments conducted inewas quantified. (g) Recombinant TDP1 or TDP1K111Rwas subjected toin vitroSUMOylation reactions in the presence of wild-type SUMO1 'WT' or mutant SUMO1 'MT' and analysed by immunoblotting. (h–j) Serial dilutions of SUMOylation reactions were subsequently mixed with Top1–DSBs (h,i) or Top1–SSBs (j) and analysed by denaturing PAGE and phosphorimaging. Reaction products were quantified relative to total labelled substrate and percentage conversion to 3′-P was quantified. Error bars, s.e.m. ofn=3 independent experiments. Figure 4: The K111R mutation does not result in a measurable change of TDP1 structure or catalytic activity. ( a ) Recombinant TDP1 or TDP1 K111R was mixed with SYPRO-Orange, and melting profiles were obtained between 20 and 70 °C using a ramping rate of 0.03 °C s −1 . Data were normalized to a fraction of protein in its denatured state and presented as normalized relative fluorescence. Melting temperatures ( T m ) were determined according to the Boltzmann model [55] . Error bars represent s.d. from n =3 independent replicates. ( b , c ) Recombinant TDP1 or TDP1 K111R was placed in a 0.2-mm quartz cuvette and the circular dichroism spectrum determined using a JASCO J-715 spectropolarimeter. Scans were performed from 260 to 195 nm, buffer baselines were subtracted, and data recorded with a high-tension voltage 'HT [V]' <550 V. Data represent the average of n =4 independent replicates±s.e.m. ( d ) Subtraction of the TDP1 K111R spectra from that of TDP1 shows no gross structural difference. ( e ) Decreasing concentrations (30, 15, 7 and 3 nM) of purified recombinant TDP1 or TDP1 K111R was incubated with a 32 P-radiolabelled duplex-nicked substrate (50 nM) harbouring a 3′-phosphotyrosine 'PY' at the nick (inset). Repair products were analysed by denaturing PAGE and phosphorimaging. Positions of the 32 P-radiolabelled substrate 'PY' and product 'P' are indicated by arrows. ( f ) Reaction products 'P' were quantified relative to total labelled substrate 'P+PY' and percentage conversion to 3′-P from experiments conducted in e was quantified. ( g ) Recombinant TDP1 or TDP1 K111R was subjected to in vitro SUMOylation reactions in the presence of wild-type SUMO1 'WT' or mutant SUMO1 'MT' and analysed by immunoblotting. ( h – j ) Serial dilutions of SUMOylation reactions were subsequently mixed with Top1–DSBs ( h , i ) or Top1–SSBs ( j ) and analysed by denaturing PAGE and phosphorimaging. Reaction products were quantified relative to total labelled substrate and percentage conversion to 3′-P was quantified. Error bars, s.e.m. of n =3 independent experiments. Full size image SUMOylation of TDP1 does not alter enzymatic activity Next, we considered the possibility that SUMOylation may alter protein function by introducing structural changes that result in changes in enzymatic activity [29] , [30] . To test this possibility, we subjected human recombinant TDP1 or TDP1 K111R to SUMOylation reactions in the presence of wild-type SUMO1 or mutant SUMO1 ( Fig. 4g ) and incubated reaction products with the synthetic Top1 substrates ( Fig. 4h–j ). We also compared the effect of SUMOylation on TDP1 produced in mammalian cells ( Fig. 5a,c,e,f ). Furthermore, we subjected purified human SUMOylated TDP1 to SENP1 treatment and compared the activity of the resulting products to that of mock-treated fractions ( Fig. 5b,d,g,h ). Incubation of Myc–TDP1 with Top1-substrate mimics resulted in a dose-dependent conversion of 3′-phosphotyrosine to 3′-phosphate, indicating that TDP1 catalytic activity was not affected by Myc, His or GFP tags. Quantification of reaction products at different concentrations or at different time points revealed no marked impact of SUMOylation on TDP1 activity ( Fig. 5e–h ). We conclude from these experiments that SUMO1 conjugation to TDP1 does not affect its enzymatic activity. We also excluded the possibility that TDP1 SUMOylation might modulate interaction with DNA ligase IIIα (Lig3α), a known binding partner and a component of the SSB repair machinery ( Fig. 6a,b ). Using western blotting, we could not detect a measurable increase of TDP1 SUMOylation after exposure to exogenous DNA damage ( Supplementary Fig. S1 ). This suggests that TDP1 SUMOylation is a housekeeping modification that occurs, as is also the case with other SUMO1-modified targets such as fission yeast Top1 and human Kap1 (refs 31 and 32 ), at low steady-state levels where cycles of conjugation and deconjugation are associated with endogenous levels of DNA breaks. Furthermore, SUMOylation did not alter TDP1 nucleolar exclusion after DNA damage, as determined by live and fixed cell fluorescence microscopy ( Fig. 6c–e ). 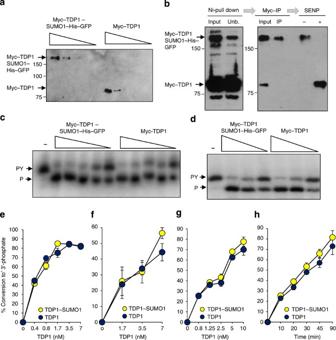Figure 5: SUMOylation of TDP1 does not display measurable impact on catalytic activity. (a) Lysates from HEK293 cells expressing Myc–TDP1 alone or additionally expressing His–GFP–SUMO1 were incubated with Ni-beads to purify His-tagged proteins, followed by Myc-immunoprecipitation. Extracts were fractionated by SDS–PAGE and 1/10 serial dilutions analysed by immunoblotting using anti-Myc antibodies. (b) Lysates from HEK293 cells expressing Myc–TDP1 and His–GFP–SUMO1 'Input' were incubated with Ni-beads, fractionated by SDS–PAGE and immunoblotted with anti-TDP1 antibodies. 'Unb.' is the unbound material. His-tagged products enriched on Ni-beads were eluted with imidazole and subjected to Myc-immunoprecipitation. The immunoprecipitate was then incubated with buffer alone '−' or buffer containing 1 μg SENP1 '+'. Purified Myc–TDP1–SUMO1–His–GFP and Myc–TDP1 were quantified by comparing with known concentrations of recombinant TDP1 analysed by immunoblotting. (c,d) Serial dilutions of Myc–TDP1 or Myc–TDP1–SUMO1–His–GFP from purifications shown in (a,b, respectively) were incubated with32P-radiolabelled Top1-substrates and reaction products analysed by denaturing PAGE and phosphorimaging. Reaction products from experiments using purification, shown ina, were quantified from Top1–DSBs (e) or Top1–SSBs (f) relative to total labelled substrate, and percentage conversion to 3′-P was calculated fromn=3 independent experiments±s.e.m. Conversion to 3′-P was determined from the purification, shown inb, at the indicated concentrations (g) or at 10 nM purified human TDP1 at the indicated time periods (h). Error bars, s.e.m ofn=3 independent experiments fromn=2 biological replicates. Figure 5: SUMOylation of TDP1 does not display measurable impact on catalytic activity. ( a ) Lysates from HEK293 cells expressing Myc–TDP1 alone or additionally expressing His–GFP–SUMO1 were incubated with Ni-beads to purify His-tagged proteins, followed by Myc-immunoprecipitation. Extracts were fractionated by SDS–PAGE and 1/10 serial dilutions analysed by immunoblotting using anti-Myc antibodies. ( b ) Lysates from HEK293 cells expressing Myc–TDP1 and His–GFP–SUMO1 'Input' were incubated with Ni-beads, fractionated by SDS–PAGE and immunoblotted with anti-TDP1 antibodies. 'Unb.' is the unbound material. His-tagged products enriched on Ni-beads were eluted with imidazole and subjected to Myc-immunoprecipitation. The immunoprecipitate was then incubated with buffer alone '−' or buffer containing 1 μg SENP1 '+'. Purified Myc–TDP1–SUMO1–His–GFP and Myc–TDP1 were quantified by comparing with known concentrations of recombinant TDP1 analysed by immunoblotting. ( c , d ) Serial dilutions of Myc–TDP1 or Myc–TDP1–SUMO1–His–GFP from purifications shown in ( a , b , respectively) were incubated with 32 P-radiolabelled Top1-substrates and reaction products analysed by denaturing PAGE and phosphorimaging. Reaction products from experiments using purification, shown in a , were quantified from Top1–DSBs ( e ) or Top1–SSBs ( f ) relative to total labelled substrate, and percentage conversion to 3′-P was calculated from n =3 independent experiments±s.e.m. Conversion to 3′-P was determined from the purification, shown in b , at the indicated concentrations ( g ) or at 10 nM purified human TDP1 at the indicated time periods ( h ). Error bars, s.e.m of n =3 independent experiments from n =2 biological replicates. 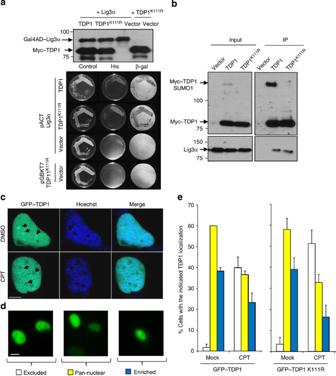Figure 6: The K111R mutation does not alter TDP1 subcellular localization or interaction with Lig3α. (a) Yeast Y190 cells harbouring pGBKT7–TDP1or pGBKT7–TDP1K111Rand pACT or pACT–Lig3αconstructs were plated onto selective media either containing 'control' or lacking 'His' histidine to test for the activation of theHis3reporter gene. Activation of theβ-Galreporter gene was determined using filter lifts from control plates. Expression levels of Myc–TDP1 or Myc–TDP1K111R(Gal4-binding domain fusion protein) and Lig3α (Gal4-activation domain fusion) were determined by immunoblotting with anti-Myc (9B11; Cell Signalling) or anti-Gal4 AD antibodies (06-283; Millipore). (b) HEK293 cells (∼4×106) were transfected with Myc–TDP1 and GFP–SUMO1, and total cell extract subjected to immunoprecipitation using anti-Myc monoclonal antibodies (9B11; Cell Signaling). Immunoprecipitates were fractionated by SDS–PAGE and analysed by immunoblotting using anti-Myc (top) or anti-Lig3α antibodies (bottom). Input is∼5% of total cell extract used. (c) Human MRC5 cells were plated onto glass-bottom dishes and transfected with pMCEGFP–TDP1. Cells were incubated with DMSO 'DMSO' or 2 μM CPT 'CPT' for 1 h at 37 °C. DNA was counterstained with Hoechst 33285, and GFP-positive cells photographed with a ×40/1.2-W objective using a Zeiss Axiovert confocal microscope. Arrowheads point at the position of nucleoli. (d,e) A549 cells transiently transfected with pMCEGFPP–TDP1'GFP–TDP1' or the SUMOylation-deficient mutant pMCEGFPP–TDP1K111R'GFP–TDP1 K111R' were mock treated 'Mock' or incubated with 30 μM CPT 'CPT' for 30 min at 37 °C. Cells were then fixed, DNA counterstained with 4,6-diamidino-2-phenylindole, and analysed with a ×60/oil objective using a Deltavision microscope. A representative images depicting cells with GFP–TDP1 excluded from nucleoli 'excluded', concentrated in nucleoli 'enriched' or exhibited pan-nuclear distribution 'Pan-nuclear' are shown ind. The average number of cells with the indicated GFP–TDP1 localization pattern was measured from a total of∼60 cells and presented as average±s.e.m. fromn=3 biological replicates; Scale bar, 10 μm. Full size image Figure 6: The K111R mutation does not alter TDP1 subcellular localization or interaction with Lig3α. ( a ) Yeast Y190 cells harbouring pGBKT7– TDP1 or pGBKT7 –TDP1 K111R and pACT or pACT– Lig3α constructs were plated onto selective media either containing 'control' or lacking 'His' histidine to test for the activation of the His3 reporter gene. Activation of the β-Gal reporter gene was determined using filter lifts from control plates. Expression levels of Myc–TDP1 or Myc–TDP1 K111R (Gal4-binding domain fusion protein) and Lig3α (Gal4-activation domain fusion) were determined by immunoblotting with anti-Myc (9B11; Cell Signalling) or anti-Gal4 AD antibodies (06-283; Millipore). ( b ) HEK293 cells ( ∼ 4×10 6 ) were transfected with Myc–TDP1 and GFP–SUMO1, and total cell extract subjected to immunoprecipitation using anti-Myc monoclonal antibodies (9B11; Cell Signaling). Immunoprecipitates were fractionated by SDS–PAGE and analysed by immunoblotting using anti-Myc (top) or anti-Lig3α antibodies (bottom). Input is ∼ 5% of total cell extract used. ( c ) Human MRC5 cells were plated onto glass-bottom dishes and transfected with pMCEGFP– TDP1 . Cells were incubated with DMSO 'DMSO' or 2 μM CPT 'CPT' for 1 h at 37 °C. DNA was counterstained with Hoechst 33285, and GFP-positive cells photographed with a ×40/1.2-W objective using a Zeiss Axiovert confocal microscope. Arrowheads point at the position of nucleoli. ( d , e ) A549 cells transiently transfected with pMCEGFPP– TDP1 'GFP–TDP1' or the SUMOylation-deficient mutant pMCEGFPP– TDP1 K111R 'GFP–TDP1 K111R' were mock treated 'Mock' or incubated with 30 μM CPT 'CPT' for 30 min at 37 °C. Cells were then fixed, DNA counterstained with 4,6-diamidino-2-phenylindole, and analysed with a ×60/oil objective using a Deltavision microscope. A representative images depicting cells with GFP–TDP1 excluded from nucleoli 'excluded', concentrated in nucleoli 'enriched' or exhibited pan-nuclear distribution 'Pan-nuclear' are shown in d . The average number of cells with the indicated GFP–TDP1 localization pattern was measured from a total of ∼ 60 cells and presented as average±s.e.m. from n =3 biological replicates; Scale bar, 10 μm. Full size image SUMOylation aids accumulation of TDP1 at sites of DNA damage We next considered the possibility that TDP1 SUMOylation might affect its local concentration at sites of DNA damage. This would be an appealing mechanism to increase substrate spectrum, as in vitro data suggest a requirement for a high concentration of TDP1 to process SSBs [16] , [23] . The difference in unrepaired SSBs that accumulate in TDP1 K111R compared with TDP1-expressing cells could be attributed to differences in the local concentration of TDP1 at sites of DNA damage ( Supplementary Fig. S2 ). To examine whether TDP1 SUMOylation fulfils this function, we compared the accumulation of GFP–TDP1 to that of GFP–TDP1 K111R at sites of ultraviolet A laser-induced DNA damage in mammalian cells. Laser damage induces a mixture of nicks, gaps, SSBs and DSBs, all of which have been shown to trap Top1, resulting in Top1–DNA breaks [33] , [34] , [35] . In addition, a subset of these breaks may be direct substrates for TDP1 (refs 7 , 12 and 36 ). While GFP–TDP1 accumulated rapidly at sites of laser damage reaching a maximum level within 5 s, accumulation of GFP–TDP1 K111R was slower and less extensive ( Fig. 7a–c ). Interestingly, accumulation of GFP–TDP1 K111R continued to increase over the entire time course of the experiment, perhaps reflecting the need to continue protein accumulation to achieve levels similar to that seen with GFP–TDP1. 90 s after DNA damage, the local enrichment of GFP–TDP1 at laser stripes was ∼ 150% compared with ∼ 125% for GFP–TDP1 K111R ( Fig. 7a ). This difference was not due to differences in TDP1 expression, as the global expression was similar by western blotting ( Fig. 7a , inset) and, more importantly, only cells that showed similar level of GFP–TDP1 total fluorescence were subjected to the tracking experiments ( Fig. 7b ). Notably, the K111R mutation did not ablate recruitment completely, suggesting that either recruitment is partially SUMOylation-dependent or other SUMO sites, although not detected biochemically, may contribute to the remaining fraction of enrichment. 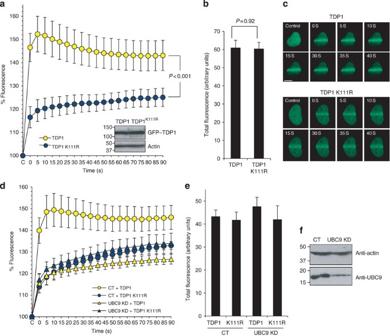Figure 7: TDP1 SUMOylation promotes its accumulation at sites of DNA damage. (a) Human MRC5 cells were plated onto glass-bottom dishes and transfected with pMCEGFP–TDP1'TDP1' or pMCEGFP–TDP1K111R'TDP1 K111R'. Cells expressing similar total GFP signal were locally irradiated with a ultraviolet A laser, and GFP–TDP1 accumulation at the site of damage was quantified for the indicated time periods (seconds), where 'C' represents undamaged and '0' the enrichment obtained immediately after damage. Data are plotted as the percentage increase in fluorescence (arbitrary units) at the site of ultraviolet A irradiation. Data are the average±s.e.m. of∼60 cells measured fromn=6 biological replicates. The difference between the accumulation of GFP–TDP1 (yellow circles) and GFP–TDP1 K111R (blue circles) was statistically significant at all time points examined (P<0.001, Student'st-test). Global expression of GFP–TDP1 was analysed by immunoblotting using anti-TDP1 antibodies, inset. (b) Average total fluorescence±s.e.m. from cells analysed inashowing comparable level of expression between GFP–TDP1 and GFP–TDP1K111R. (c) Representative images of cells from experiments presented inaare shown before irradiation 'control', immediately after '0 s' and at the indicated time points '5–40 s'. Scale bar, 10 μm. (d) MRC5 cells were transfected with non-silencing control constructs 'CT' or with constructs encoding short hairpin RNA toUBC9'UBC9 KD' and stable cells were subsequently transfected with pMCEGFP–TDP1'TDP1' or with pMCEGFP–TDP1K111R'TDP1 K111R'. Cells expressing similar total GFP signal were locally irradiated with an ultraviolet A laser, and GFP–TDP1 accumulation at the site of DNA damage was quantified as described ina. Data are the mean±s.e.m. of∼40 cells measured fromn=3 biological replicates. (e) Average total fluorescence±s.e.m. from cells analysed indshowing no difference in expression levels between GFP–TDP1 and GFP–TDP1K111R. (f) Lysate from control 'CT' or UBC9-depleted 'UBC9 KD' cells were fractionated by SDS–PAGE and analysed by immunoblotting using anti-UBC9 (Abcam) or anti-actin antibodies. Figure 7: TDP1 SUMOylation promotes its accumulation at sites of DNA damage. ( a ) Human MRC5 cells were plated onto glass-bottom dishes and transfected with pMCEGFP– TDP1 'TDP1' or pMCEGFP– TDP1 K111R 'TDP1 K111R'. Cells expressing similar total GFP signal were locally irradiated with a ultraviolet A laser, and GFP–TDP1 accumulation at the site of damage was quantified for the indicated time periods (seconds), where 'C' represents undamaged and '0' the enrichment obtained immediately after damage. Data are plotted as the percentage increase in fluorescence (arbitrary units) at the site of ultraviolet A irradiation. Data are the average±s.e.m. of ∼ 60 cells measured from n =6 biological replicates. The difference between the accumulation of GFP–TDP1 (yellow circles) and GFP–TDP1 K111R (blue circles) was statistically significant at all time points examined ( P <0.001, Student's t -test). Global expression of GFP–TDP1 was analysed by immunoblotting using anti-TDP1 antibodies, inset. ( b ) Average total fluorescence±s.e.m. from cells analysed in a showing comparable level of expression between GFP–TDP1 and GFP–TDP1 K111R . ( c ) Representative images of cells from experiments presented in a are shown before irradiation 'control', immediately after '0 s' and at the indicated time points '5–40 s'. Scale bar, 10 μm. ( d ) MRC5 cells were transfected with non-silencing control constructs 'CT' or with constructs encoding short hairpin RNA to UBC9 'UBC9 KD' and stable cells were subsequently transfected with pMCEGFP– TDP1 'TDP1' or with pMCEGFP– TDP1 K111R 'TDP1 K111R'. Cells expressing similar total GFP signal were locally irradiated with an ultraviolet A laser, and GFP–TDP1 accumulation at the site of DNA damage was quantified as described in a . Data are the mean±s.e.m. of ∼ 40 cells measured from n =3 biological replicates. ( e ) Average total fluorescence±s.e.m. from cells analysed in d showing no difference in expression levels between GFP–TDP1 and GFP–TDP1 K111R . ( f ) Lysate from control 'CT' or UBC9-depleted 'UBC9 KD' cells were fractionated by SDS–PAGE and analysed by immunoblotting using anti-UBC9 (Abcam) or anti-actin antibodies. Full size image If it is true that TDP1 SUMOylation promotes repair by facilitating its accumulation at sites of DNA damage, then depletion of UBE2I (UBC9), the obligate SUMO-conjugating enzyme, should similarly reduce accumulation of TDP1 at sites of DNA damage. To test this, we depleted UBC9 in MRC5 cells using short hairpin RNA and compared the accumulation of GFP–TDP1. As predicted, depletion of UBC9 led to a marked reduction of the ability of GFP–TDP1 to accumulate at sites of laser damage ( Fig. 7b–f ). Enrichment of GFP–TDP1 in UBC9-depleted cells displayed similar dynamics to that of GFP–TDP1 K111R , as it continued to increase during the time course of the experiment. Importantly, depletion of UBC9 did not result in further reduction in the accumulation of GFP–TDP1 K111R , indicating that the observed effect was due to SUMOylation. Taken together, these results indicate that SUMOylation of TDP1 at K111 facilitates its accumulation at sites of DNA damage, thereby enhancing its DNA repair capacity. Contribution to the repair of transcription-associated SSBs A major source of Top1-breaks is the collision of Top1 intermediates with elongating RNA polymerases during transcription. Inhibiting RNA polymerase II by 5,6-dichlorobenzimidazole 1-b- D -ribofuranoside (DRB) or α-amanitin has been shown to reduce the extent of CPT-induced DNA SSBs [4] , [37] . We reasoned that if TDP1 SUMOylation contributes to its recruitment to sites of transcription-associated SSBs, then inhibiting transcription should result in reduced accumulation of TDP1. Consistent with this prediction, pretreatment of GFP–TDP1-expressing cells with the transcription inhibitor DRB led to reduction in TDP1 accumulation at sites of laser damage ( Fig. 8a,b ). The reduction in recruitment was less than that observed for mock-treated GFP–TDP K111R , which could reflect a role for TDP1 SUMOylation during damage generated by DRB-resistant RNA polymerases. Alternatively, it could be due to roles for TDP1 SUMOylation unrelated to transcription. Importantly, DRB did not affect the initial recruitment of GFP–TDP1 K111R , suggesting a role for TDP1 SUMOylation at K111 during the repair of transcription-blocking lesions. However, DRB ablated the time-dependent increase of GFP–TDP1 K111R accumulation during the subsequent 90-s observation period. We reason that inhibiting transcription may reduce the frequency of collision of Top1 intermediates with elongating RNA polymerase II, thereby reducing the need for recruiting more GFP–TDP1 K111R . We next quantified the extent of transcription-associated SSBs using alkaline comet assays. For these experiments, we used HEK293 cells to achieve ∼ 90% transfection efficiency. If the difference in repair capacity observed between TDP1 and TDP1 K111R was, at least in part, due to a role for TDP1 SUMOylation in repairing transcription-associated SSBs, then inhibiting transcription should ablate or reduce this difference. While cells expressing TDP1 K111R accumulated a higher level of SSBs compared with TDP1 expressing cells, they both decreased to a comparable level following incubation with DRB ( Fig. 8c,d ; P =0.78; t -test), suggesting that TDP1 SUMOylation contributes to the repair of transcription-associated SSBs. Taken together, these data suggest that TDP1 SUMOylation at K111 participates in the overall repair of transcription-dependent SSBs. 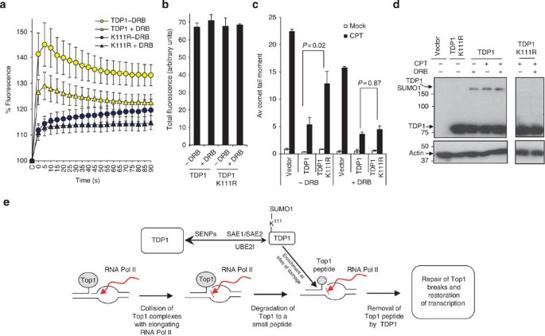Figure 8: Accumulation of TDP1 at sites of DNA damage is in part transcription dependent. (a) MRC5 cells expressing GFP–TDP1 or GFP–TDP1 K111R were incubated with DMSO '-DRB' or with 50 μM 5,6-dichlorobenzimidazole 1-b-D-ribofuranoside '+DRB' for 2 h at 37 °C. Cells expressing similar total GFP signal were irradiated with an ultraviolet A laser, and GFP–TDP1 accumulation at the site of damage was quantified. Data are the mean±s.e.m. of∼40 cells fromn=4 biological replicates. Note that the difference between the accumulation of GFP–TDP1 in the absence (yellow circles) and presence (yellow triangles) of DRB was statistically significant (P<0.05, Student'st-test). (b) Average total fluorescence±s.e.m. for cells analysed ina. (c) HEK293 cells were transfected with empty vector 'vector', Myc–TDP1 'TDP1' or Myc–TDP1K111R'TDP1 K111R' and GFP–SUMO1. Cells were incubated with DMSO 'mock' or treated with 50 μM camptothecin 'CPT' with or without previous incubation with 50 μM DRB for 2 h. DNA strand breakage was quantified by alkaline comet assays and presented as mean tail moment. Data are the average±s.e.m. fromn=3 biological replicates, where 50 cells per sample were blindly scored from each experiment. Statistical analyses (Student'st-test) were conducted to compare the difference between TDP1 and TDP1 K111R in the absence or presence of DRB, and the correspondingP-values are depicted. (d) Lysate from cells used for experiments incwere fractionated by SDS–PAGE and analysed by immunoblotting. (e) Collision of elongating RNA polymerases, such as RNA Pol II with Top1 intermediates, leads to stalling of the polymerase with subsequent proteasomal degradation of Top1, and possibly the stalled RNA Pol. We propose that these collision events recruit TDP1 to sites of polymerase stalling. TDP1 exists in equilibrium between unmodified (the majority) and a SUMOylated version (a tiny proportion), and the balance is maintained by the opposing activities of SUMO conjugation (SAE1/2, UBC9 and possibly a SUMO ligase) and deconjugation (SENPs). We show that TDP1 SUMOylation occurs primarily at K111 and propose that SUMOylated TDP1 is at least, in part, engaged in dealing with the transcription-blocking lesions. Figure 8: Accumulation of TDP1 at sites of DNA damage is in part transcription dependent. ( a ) MRC5 cells expressing GFP–TDP1 or GFP–TDP1 K111R were incubated with DMSO '-DRB' or with 50 μM 5,6-dichlorobenzimidazole 1-b- D -ribofuranoside '+DRB' for 2 h at 37 °C. Cells expressing similar total GFP signal were irradiated with an ultraviolet A laser, and GFP–TDP1 accumulation at the site of damage was quantified. Data are the mean±s.e.m. of ∼ 40 cells from n =4 biological replicates. Note that the difference between the accumulation of GFP–TDP1 in the absence (yellow circles) and presence (yellow triangles) of DRB was statistically significant ( P <0.05, Student's t -test). ( b ) Average total fluorescence±s.e.m. for cells analysed in a . ( c ) HEK293 cells were transfected with empty vector 'vector', Myc–TDP1 'TDP1' or Myc–TDP1 K111R 'TDP1 K111R' and GFP–SUMO1. Cells were incubated with DMSO 'mock' or treated with 50 μM camptothecin 'CPT' with or without previous incubation with 50 μM DRB for 2 h. DNA strand breakage was quantified by alkaline comet assays and presented as mean tail moment. Data are the average±s.e.m. from n =3 biological replicates, where 50 cells per sample were blindly scored from each experiment. Statistical analyses (Student's t -test) were conducted to compare the difference between TDP1 and TDP1 K111R in the absence or presence of DRB, and the corresponding P -values are depicted. ( d ) Lysate from cells used for experiments in c were fractionated by SDS–PAGE and analysed by immunoblotting. ( e ) Collision of elongating RNA polymerases, such as RNA Pol II with Top1 intermediates, leads to stalling of the polymerase with subsequent proteasomal degradation of Top1, and possibly the stalled RNA Pol. We propose that these collision events recruit TDP1 to sites of polymerase stalling. TDP1 exists in equilibrium between unmodified (the majority) and a SUMOylated version (a tiny proportion), and the balance is maintained by the opposing activities of SUMO conjugation (SAE1/2, UBC9 and possibly a SUMO ligase) and deconjugation (SENPs). We show that TDP1 SUMOylation occurs primarily at K111 and propose that SUMOylated TDP1 is at least, in part, engaged in dealing with the transcription-blocking lesions. Full size image Top1-linked DNA breaks underlie the clinical utility of an important class of anticancer drugs, and their progressive accumulation causes neurodegeneration in humans [1] , [38] , [39] , [40] . A key factor in the repair of Top1-breaks is TDP1, mutation of which causes the demise of postmitotic tissue. Here we report that TDP1 is a substrate for SUMO modification, which occurs primarily at lysine 111 within the vertebrate-conserved N-terminal domain. SUMOylation promotes accumulation of TDP1 at sites of DNA damage, thereby accelerating the rate of SSB repair and contributes, at least in part, to the repair of transcription-generated SSBs, the major source of Top1-breaks in non-cycling cells. These observations raise the possibility of an important regulatory role in postmitotic tissue. Notably, ∼ 4-fold difference in the rapid clearance of SSBs results in severe neurological dysfunction in murine model systems [22] and has been linked to ataxia in humans [1] , [41] , [42] . Collision of elongating RNA polymerase II with Top1 intermediates results in stalling of transcription and triggers partial degradation of Top1 to a small peptide [43] . TDP1 can then access these structures to remove the stalled Top1 peptide from DNA termini [23] , [44] . We propose that collision with RNA polymerases is a trigger to degrade Top1 and to subsequently enrich TDP1 at sites of DNA damage ( Fig. 8e ). The latter process is, at least in part, dependent on SUMOylation of TDP1 at lysine 111. We propose a further, evolutionarily conserved, layer of regulation via a SUMO–SIM interaction that maintains TDP1 at sites of DNA damage. There is precedence for the involvement of SUMO during Top1 repair. Top1 itself, the main source of DNA breaks that require TDP1, is also a substrate for SUMO conjugation [45] , [46] . In fission yeast, the SUMO conjugation machinery also has a role for dealing with Top1-breaks [47] . The Nse2 E3 SUMO ligase functions together with the fission yeast structure-specific nuclease Rad16-Swi10 to facilitate the repair of Top1-breaks, independently of Tdp1 (refs 32 and 48 ). Notably, lysine 111 is absent in fission yeast Tdp1, highlighting an evolutionarily driven SUMO regulation for human TDP1. Mutation of the SUMO acceptor lysine 111 to arginine did not result in an apparent impact on the core structure of TDP1, as indicated by the thermal shift profiles, circular dichroism spectrograms and by comparing enzymatic activities of the recombinant proteins. While CD spectra showed no significant change in α-helical or β-sheet content, it pointed at a possible minor change in conformation, which is unlikely to be of biological relevance, as enzymatic activities was not affected. Moreover, cellular TDP1 and TDP1 K111R interacted to the same extent with Lig3α, which is known to bind to that domain [17] , [18] , as measured by two independent assay methods ( Fig. 6 ). Knockdown of UBC9 reduced recruitment of TDP1 to a level similar to that of TDP1 K111R , but had no impact on TDP1 K111R recruitment, indicating that the difference was due to SUMOylation. Furthermore, overexpression of SUMO1 facilitated repair of cells expressing TDP1, but not TDP1 K111R , further supporting that the observed phenotype was due to SUMOylation. Crystal structure, cell-free and DNA binding studies suggest that high local concentrations of TDP1 are required to process Top1–SSBs [16] , [49] , [50] . However, how vertebrate cells achieve this was not clear [5] , [16] , [51] . Here we examined whether SUMOylation of TDP1 increased its catalytic activity, using the 3′-phosphotyrosine substrate to mimic Top1-linked DNA breaks. SUMOylated TDP1 prepared in vitro or purified from mammalian cells exhibited similar catalytic activity to the unSUMOylated version. It is possible that SUMOylation facilitates binding of Top1 peptide to the peptide-binding pocket of TDP1 and thus increases catalytic activity when using a peptide substrate instead of a phosphotyrosine substrate. However, we do not favour this possibility, as the peptide-binding pocket is distant form the SUMOylation site. Instead, our results show that SUMOylation promotes TDP1 accumulation at sites of DNA damage, ensuring sufficiently rapid and proficient repair of SSBs ( Figs 7 and 8 ). SUMOylation has been previously implicated in concentrating enzymatic activities and triggering the formation of nuclear assemblies, such as PML bodies [52] , [53] however, it has not been linked to repair of SSBs, a highly abundant form of endogenous DNA damage and a major threat to genome integrity. Notably, we observed that persistent overexpression of TDP1, but not the SUMOylation-defective mutant, was poorly tolerated in mammalian cells. This is likely due to the efficient accumulation of TDP1 at damaged sites with subsequent generation of excessive 3′-phosphate termini that require further processing by limiting downstream factors such as PNK [54] . Thus, SUMOylation appears to target specifically a subset of TDP1 to promote sufficiently rapid turnover of endogenous Top1–SSBs. It is not known at what level Top1-breaks arise in cells. However, the fact that they do arise in the absence of exogenous DNA damage is suggested by the progressive degeneration of the cerebellum of patients with defective TDP1 and by experiments in fission yeast where depletion of Tdp1 and parallel pathways led to the generation of Top1-breaks [1] , [32] . Thus, devising efficient mechanisms to deal with endogenous Top1-breaks is critical for the maintenance of genetic integrity, particularly in postmitotic tissue. In summary, we report here that human TDP1 is SUMOylated at lysine 111 and that SUMOylation promotes its accumulation at sites of damaged DNA, thereby facilitating the repair of SSBs. These data identify a molecular role for SUMOylation during TDP1-mediated SSB repair reactions and implicates this process in protecting postmitotic tissue from genotoxic stress. Yeast two-hybrid screen and analyses Sacharomyces cerevisiae Y190 cells (Clontech) were transformed with pGBKT7– TDP1 S81E , and transformants were plated onto minimal media plates (glucose and yeast nitrogen base without amino acids) additionally containing adenine, histidine and leucine. Pooled populations of transformants were streaked and single clones picked to ensure good expression of the fusion proteins. Y190 cells expressing pGBKT– TDP1 S81E were transformed with 16 μg of pACT human cDNA library and transformants plated onto minimal media supplemented with adenine and 50 mM 3-amino-1,2,4-triazole (3AT), but lacking leucine, tryptophan and histidine (His-). The activation of the His reporter gene was indicated by growth on His- plates after 4–7 days at 30 °C. A total number of 5×10 6 clones were screened, as estimated from the transformation efficiency on minimal media plates with adenine and histidine. Healthy-looking colonies were isolated, rescreened for growth on His- plates. Potential clones were tested for the activation of the β-Gal reporter by qualitative X-Gal (5-bromo-4-chloro-3-indolyl-β- D -galacto-pyranoside) assays on colony filter lifts from control plates. Following confirmation of positive clones, the corresponding pACT constructs were isolated and subjected to sequencing. We identified 14 independent clones encoding full-length human UBE2I according to the published DNA sequence (NM_003345). Antibodies used for the detection of fusion proteins are listed in Supplementary Methods . Cell-free SUMOylation assays The generation and purification of recombinant proteins and their quantification are detailed in Supplementary Methods . Purified His–TDP1 or His–TDP1 mutants (430 nM) were incubated with purified SAE1/SAE2 (50 nM), UBC9 (500 nM), SUMO1, SUMO2 or SUMO3 (30 μM) in 50 mM Tris–HCl, pH 8.0; 50 mM NaCl, 5 mM MgCl 2 , 10% glycerol, 0.5 mM DTT and 5 mM ATP (Activemotif). Reactions were incubated at 30 °C for 3 h unless otherwise indicated, followed by fractionation on SDS–PAGE and analyses by western blotting using anti-SUMO1, anti-SUMO2/3, anti-p53 (Activemotif, 1:3,000) or anti-TDP1 polyclonal antibodies (ab4166; Abcam, 1:2,000). Note that we noticed a nonspecific binding of the anti-SUMO1 antibodies (Activemotif) to unmodified SUMO1 targets. To confirm that the modification is in fact for SUMO1, we also used anti-SUMO1 monoclonal antibodies from Santa Cruz (clone 0–11; SC-5308, 1:2,000). While both antibodies recognized the same SUMOylated species, the latter did not pick up the unmodified protein. Circular dichroism spectroscopy Recombinant proteins were dialysed in 30 mM sodium phosphate buffer, pH 7.4, and filtered immediately before the spectrum was obtained through 0.2-micron filters (Millipore). The concentration of recombinant proteins was accurately determined immediately before, during and after the CD scans, to ensure accurate secondary structure estimations. Samples were normalized to the lowest concentration (0.6 mg ml −1 ), placed in a 0.2-mm quartz cuvette (Starna, Essex, UK) and measurements taken using a JASCO J-715 spectropolarimeter (JASCO). The CD spectrum of the buffer alone was subtracted from that of the sample, and time constant was set to 4 s with a scan rate at 50 nm min −1 . The bandwidth was 1 nm and the sensitivity set to standard. Scans were performed from 260 to 190 nm with a 0.1-nm data pitch and continuous scan mode. A Peltier device was used to maintain a temperature at 10 °C. The buffer baselines were subtracted and data represent the average of four independent experiments±s.e.m. Immunoprecipitation The generation and maintenance of mammalian cells are provided in Supplementary Methods . HEK293 ( ∼ 1.5×10 6 ) cells were transfected using standard calcium phosphate precipitation, and 2 days later, cells were lysed in 200 μl lysis buffer (20 mM HEPES pH7.4, 0.5% NP40, 40 mM NaCl, 2 mM MgCl 2 , 1× protease inhibitor cocktail (Roche) 1× phosphatase inhibitor cocktail (Roche), 20 mM N -ethyl maleimide, 25 U ml −1 benzonase (Merck)). Lysates were incubated for 30 min on ice, cleared by centrifugation at 13,000 r.p.m. for 10 min, and NaCl concentration adjusted to either 150 mM for coimmunoprecipitation to examine protein–protein interaction or 300 mM to detect in vivo SUMOylation. Anti-Myc antibodies (9B11; Cell Signaling) were added to the lysate at 1 μl per 200 μl lysate volume and the mixture was rotated at 4 °C for 1 h. Following centrifugation at 13,000 r.p.m. for 10 min, supernatant was then added to protein-G sepharose beads (Sigma), followed by rolling at 4 °C for 1 h. Beads were washed three times with wash buffer (20 mM HEPES, pH 7.4, 150 mM or 300 mM NaCl) and then resuspended in SDS loading buffer for analyses by immunoblotting. Purification of SUMOylated TDP1 from human cells Approximately 1×10 7 HEK293 cells were transfected with plasmids encoding GFP–His–SUMO1 and Myc–TDP1 and lysed, as described above, using 2× protease inhibitors and 30 mM imidazole in both the lysis and wash buffer. Following washing, SUMOylated proteins were eluted from the beads using three consecutive elutions with lysis buffer containing 250 mM imidazole. Elution fractions were pooled and SUMOylated TDP1 was purified using Myc-immunoprecipitation, as described above. Beads enriched with SUMOylated TDP1 were finally suspended in an equal volume of wash buffer. Where indicated, 80 μl bead suspension enriched with purified Myc–TDP1–SUMO1 was resuspended in 150 mM NaCl, 50 mM Tris, pH 7.5, 0.5 mM DTT. A volume of 40 μl bead suspension was then mock-treated or incubated with 0.2–1 μg of human sentrin/SUMO-specific protease-1 (SENP1; Enzo Life Sciences) for 20 min at 37 °C. Following three consecutive washes with 150 mM NaCl, 50 mM Tris, pH 7.5, beads were subjected to in vitro activity assays or analysed by immunoblotting with anti-TDP1 or anti-Myc antibodies. Quantification of purified Myc–TDP1 and Myc–TDP1–SUMO1–His–GFP was conducted by comparing with known concentrations of recombinant His–TDP1 by western blotting. The latter was determined by Bradford assays, and by comparing with Coomassie-stained BSA standards. We estimate 2 ng μl −1 bead suspension of purified human Myc–TDP1 or Myc–TDP1–SUMO1–His–GFP. Cell-free DNA repair assays Purified recombinant proteins were subjected to in vitro SUMOylation reactions and the appropriate dilutions were mixed with 50 nM 32 P-labelled oligonucleotide duplexes (see Supplementary Methods for DNA sequence) in 8 μl total volume in 25 mM HEPES, pH 8.0, 130 mM KCl and 1 mM DTT. Purified SUMOylated TDP1 from mammalian cells was quantified as described above and serial dilutions of beads were mixed with 50 nM 32 P-labelled substrates. Reactions were incubated for 1 h at 37 °C, terminated by formamide loading buffer, fractionated by denaturing PAGE, and analysed by phosphorimaging. Cellular SSB repair assays HEK293 cells or Tdp1 −/− MEFs containing empty vector or vectors expressing wild-type TDP1, TDP1 K111R or GFP–SUMO1 were subjected to 20 μM CPT (MEFs) or 50 μM CPT (HEKs) for 30 min at 37 °C, or exposed to 20 Gy IR (caesium 137, Cammael 1000) on ice. Where indicated, cells were subsequently incubated in drug-free media for the indicated repair periods. DNA strand breakage was quantified by alkaline comet assays as described in Supplementary Methods . Clonogenic survival and viability assays Following confirmation of expression by anti-TDP1 western blotting, Tdp1 −/− MEFs complemented with empty vector or with vectors expressing wild-type TDP1 or TDP1 K111R were plated in duplicate into 10-cm dishes ( ∼ 2,000 cells; untreated, 6,000 cells; CPT doses 2.5 and 5 μM, and ∼ 10,000 cells; CPT doses 7.5 and 10 μM) and incubated at 37 °C for at least 8 h. Cells were then mock-treated or treated with the indicated doses of CPT for 1 h at 37 °C. Cells were washed with PBS (3×) and then incubated for 7–10 days in drug-free medium to form macroscopic colonies. Colonies were fixed using 90% ethanol and stained with 1% methylene blue. Survival was calculated by dividing the average number of colonies on treated plates by the average number of colonies on untreated plates. Cortical neural cells were grown to confluency at 20% oxygen to elevate the oxidative load and then deprived from growth factors for 3 days, followed by electroporation with GFP–TDP1 or GFP–TDP1 K111R using Neon transfection system, according the manufacturer's instructions (Invitrogen). Cells maintained at high oxygen were exposed to fractionated pulses of 30 μM CPT (4× 30 min pulse every 3 h), and viability of GFP-positive cells was quantified from blindly coded slides using propidium iodide (Sigma) exclusion. Laser microirradiation Exponentially growing human MRC5 cells were plated onto 35-mm glass-bottom dishes (MatTek) and transfected with pMCEGFP– TDP1 or pMCEGFP– TDP1 K111R using GeneJuice (Novagen), according to the manufacturer's protocol. Twenty-four hours following transfection, cells were incubated with 10 μg ml −1 Hoechst 33285 (Sigma) for 1 h at 37 °C before irradiation. Where indicated, cells were additionally incubated with DMSO or 50 μM DRB for 2 h before irradiation. Cells expressing similar total GFP signal were irradiated with a 351-nm ultraviolet A (4.36 J m −2 ) laser channelled through a ×40/1.2-W objective using a Zeiss ConfoCor 2/LSM510 combi meta point scanning confocal microscope (Zeiss). Ultraviolet A was focused to an area of approximately 12 μm×0.1 μm, and images were captured at 5-s intervals following laser damage and quantified by ImageJ and LSM 520 Meta software. How to cite this article: Hudson, J.J.R. et al . SUMO modification of the neuroprotective protein TDP1 facilitates chromosomal single-strand break repair. Nat. Commun. 3:733 doi: 10.1038/ncomms1739 (2012).